Photovoltaic effect in few-layer black phosphorus PN junctions defined by local electrostatic gating In conventional photovoltaic solar cells, photogenerated carriers are extracted by the built-in electric field of a semiconductor PN junction, defined by ionic dopants. In atomically thin semiconductors, the doping level can be controlled by the field effect, enabling the implementation of electrically tunable PN junctions. However, most two-dimensional (2D) semiconductors do not show ambipolar transport, which is necessary to realize PN junctions. Few-layer black phosphorus (b-P) is a recently isolated 2D semiconductor with direct bandgap, high mobility, large current on/off ratios and ambipolar operation. Here we fabricate few-layer b-P field-effect transistors with split gates and hexagonal boron nitride dielectric. We demonstrate electrostatic control of the local charge carrier type and density in the device. Illuminating a gate-defined PN junction, we observe zero-bias photocurrents and significant open-circuit voltages due to the photovoltaic effect. The small bandgap of the material allows power generation for illumination wavelengths up to 940 nm, attractive for energy harvesting in the near-infrared. In the past few years, the research effort on 2D materials has rapidly increased, driven by the great variety of layered materials and their exceptional properties when reduced to a few atomic layers [1] , [2] , [3] . Owing to their remarkable mechanical [4] , [5] , electrical [6] , [7] and optical properties [8] , [9] , [10] they have proven to be promising candidates for many applications such as mass sensing [11] , transistor operation [7] , optical communication [12] and photodetection [13] , [14] , [15] , [16] . The field of electronics now has access to a large library of 2D materials, ranging from elemental gapless semiconductors (graphene), semiconducting and superconducting chalcogenides (for example, transition metal dichalcogenides) to large bandgap insulators (for example, hexagonal boron nitride, h-BN). The combined use of their exceptional properties has recently been made possible because of advancements in transfer techniques [6] , [17] , [18] . Different 2D materials can now be used as components of a single device such as a field-effect transistor, where a gate dielectric and a semiconducting channel material are needed. Owing to its atomically flat surface and its disorder-free interface with other 2D materials, h-BN is well suited to be used as a gate dielectric material [6] , [19] , [20] . Few-layer black phosphorus (b-P), a recently isolated 2D material, has shown promising characteristics for its use as channel material, such as high mobility, good current ON/OFF ratios and ambipolarity [21] , [22] , [23] , [24] , [25] , [26] , [27] , [28] . Especially the ambipolarity and the direct bandgap (optimum for visible and near-infrared (NIR) applications) make b-P an interesting candidate for electrostatically tuneable optoelectronic devices. Here we transfer h-BN and few-layer b-P on a pair of local gates to define PN junctions. The electrostatic control of the charge carrier type in different regions of a few-layer b-P flake allows us to tune the electronic behaviour from metallic to diode-like. Under illumination, the PN junctions show photovoltaic effect, demonstrating that a large internal electric field can be obtained by local gating. Beyond fabricating a locally gated PN junction based on a van der Waals heterostructure of 2D materials, our results set the ground for further research towards photodetection and energy harvesting based on few-layer b-P devices. Fabrication of locally gated b-P devices To efficiently control the doping level in different regions of the b-P flake, we fabricate a pair of local gates (Ti/AuPd, 5 nm/25 nm) separated by a 300-nm gap on a SiO 2 /Si substrate by standard e-beam lithography and metal deposition techniques ( Fig. 1a ). The schematics below each panel of Fig. 1 show a cross-section of the device after each fabrication step. On top of the local gates, we first transfer a thin (~20 nm) h-BN flake for use as gate dielectric ( Fig. 1b ). We select, by optical inspection, h-BN flakes free of large wrinkles and folds that could hamper subsequent transfer and fabrication steps. Then, we transfer a few-layer (~6–7 nm) b-P flake on top of h-BN such that it is well centred with respect to the local gates ( Fig. 1c ). Both transfer steps are performed via a recently developed deterministic dry transfer method [18] . The b-P flake is then contacted with two leads (Ti/Au 2 nm/60 nm), fabricated by e-beam lithography, metal deposition and lift-off ( Fig. 1d ). All electrical measurements are performed in a probe station in vacuum (10 −5 mbar) to minimize degradation of the b-P flakes under ambient conditions [24] , [29] . 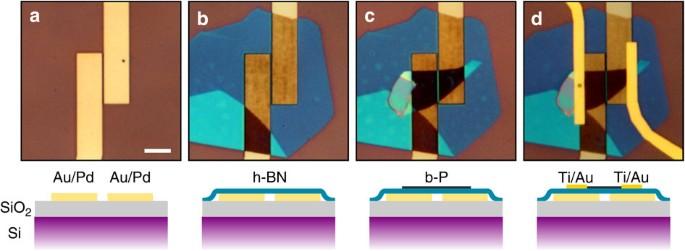Figure 1: Optical images of the fabrication of a locally gated h-BN/b-P PN junction. (a) Local gates (Au/Pd) patterned on the surface of a SiO2/Si substrate. The gap between the gates is 300-nm wide. (b) After the transfer of a thin h-BN flake on top of the split gates. (c) After the transfer of a thin b-P flake on top of the h-BN and the split gate region. (d) The final device after fabrication of the contacts (Ti/Au). The schematics below each panel show a cross-section of the device after each fabrication step. The scale bar is 5 μm for all panels. Figure 1: Optical images of the fabrication of a locally gated h-BN/b-P PN junction. ( a ) Local gates (Au/Pd) patterned on the surface of a SiO 2 /Si substrate. The gap between the gates is 300-nm wide. ( b ) After the transfer of a thin h-BN flake on top of the split gates. ( c ) After the transfer of a thin b-P flake on top of the h-BN and the split gate region. ( d ) The final device after fabrication of the contacts (Ti/Au). The schematics below each panel show a cross-section of the device after each fabrication step. The scale bar is 5 μm for all panels. 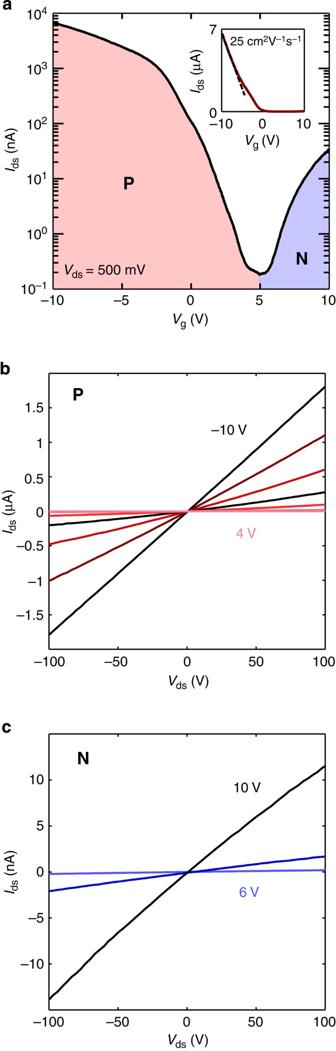Figure 2: Electrical characterization of the locally gated h-BN/b-P heterostructure. (a) Transfer characteristic atVds=500 mV. The inset shows the data in linear scale. (b) Output characteristics forVgfrom −10 to 4 V in steps of 2 V. (c) Output characteristics forVgfrom 6 to 10 V in steps of 2 V. Full size image Transistor operation of locally gated b-P Figure 2a shows the electrical transfer characteristics of a locally gated b-P flake; the source-drain current ( I ds ) is recorded at constant source-drain bias ( V ds ), while the two local gates act as a single back-gate ( V lg =V rg =V g ). The inset shows the data on a linear scale. The source-drain current is strongly modulated as V g is swept from negative to positive voltages: I ds varies from a few μA at V g =−10 V to a minimum of ~100 pA at V g =5 V and increases to tens of nA for larger V g values. The non-monotonic transfer curve is a clear signature of ambipolar transport, indicating that both hole and electron doping can be achieved, as expected for few-layer b-P [26] , [29] . From Fig. 2a , we derive that the b-P transistor on h-BN is naturally P-doped with an unintentional doping level larger than devices fabricated on SiO 2 (refs 21 , 22 , 23 , 24 , 25 , 26 , 29 ). The field-effect mobility is in the order of 25 cm 2 V −1 s −1 and the current modulation is more than a factor 10 4 for holes (0.12 cm 2 V −1 s −1 and 10 2 for electrons). We observe similar behaviour in three fabricated locally gated b-P devices. While the results shown in the main text correspond to the same device, the reader can find the characterization and data sets for the other devices in the Supplementary Figs 1–3 . Interestingly, the current values in the hole- and electron-doped regimes at the same carrier concentration differ less than one order of magnitude for all devices. This stronger ambipolar behaviour is most likely due to a more efficient gate coupling provided by the high quality (that is, high breakdown voltage) of the ultrathin h-BN ( Supplementary Fig. 4 ). Figure 2: Electrical characterization of the locally gated h-BN/b-P heterostructure. ( a ) Transfer characteristic at V ds =500 mV. The inset shows the data in linear scale. ( b ) Output characteristics for V g from −10 to 4 V in steps of 2 V. ( c ) Output characteristics for V g from 6 to 10 V in steps of 2 V. Full size image Figure 2b,c shows the conductance of the device in P- and N-type operations, respectively. The measured I ds – V ds curves are linear for both operation modes over a wide range of gate voltages, indicating that the Schottky barriers do not dominate the transport and that the Ti/Au leads make good ohmic contact to the b-P flake. The current in the hole-doped regime is higher than in the electron-doped regime, indicating that the Fermi level of the contacts is closer to the valence band than the conduction band of b-P, similar to previous devices contacted with the same metals [26] . PN junction operation of locally gated b-P The multiple gates in our device allow us not only to make an ambipolar transistor, such as in Fig. 2a , but also to locally induce hole and electron doping in different parts of the channel. 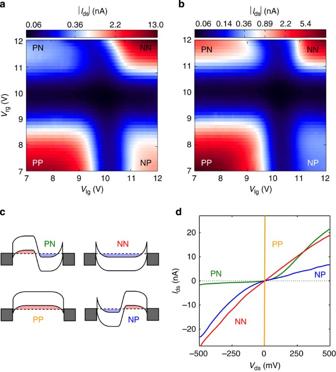Figure 3: Electrostatic control of the few-layer black phosphorus PN junction. (a) False-colour map of the magnitude of the source-drain current at constant bias voltage (+100 mV) as the voltage on the two local gates is changed independently. (b) False-colour map of the magnitude of the source-drain current at constant bias voltage (−100 mV) as the voltage on the two local gates is changed independently. (c) Band diagrams corresponding to the different device configurations. (d) Output characteristics of the device in different gate configurations (PP:Vlg=Vrg=−10 V, NN:Vlg=Vrg=10 V, NP:Vlg=10 V,Vrg=−10 V, PN:Vlg=−10 V,Vrg=10 V). Figure 3a,b show false-colour maps of the magnitude of I ds at a fixed bias voltage as the split gates are independently swept from 7 to 12 V. The gate voltage values are chosen to be close to the flatband condition as determined from the transfer characteristics measured in single back-gate configuration ( Fig. 2a ). In both maps, it is possible to distinguish four distinct regions where current flows, separated by regions where only a small current is measured (the OFF state of the device). The previously reported effect of gate-induced stress for devices on SiO 2 is drastically reduced by choosing a h-BN flake as gate dielectric that provides a more stable dielectric environment ( Supplementary Fig. 4 ). Moreover, the shift in the gate voltage is constant over several days, in contrast with the much shorter time scales (minutes) of devices fabricated on SiO 2 (ref. 26 ). Figure 3: Electrostatic control of the few-layer black phosphorus PN junction. ( a ) False-colour map of the magnitude of the source-drain current at constant bias voltage (+100 mV) as the voltage on the two local gates is changed independently. ( b ) False-colour map of the magnitude of the source-drain current at constant bias voltage (−100 mV) as the voltage on the two local gates is changed independently. ( c ) Band diagrams corresponding to the different device configurations. ( d ) Output characteristics of the device in different gate configurations (PP: V lg = V rg =−10 V, NN: V lg = V rg =10 V, NP: V lg =10 V, V rg =−10 V, PN: V lg =−10 V, V rg =10 V). Full size image The cross of suppressed conductance allows us to identify four distinct regions of doping, indicating the good control of the gates over the doping type and concentration in the b-P flake. In Fig. 3a , the NN ( V lg = V rg =12 V) and PP ( V lg = V rg =7 V) quadrants show the highest current values, as expected from the transfer characteristics in Fig. 2a . On the other hand, the measured current in the NP ( V rg =7 V, V lg =12 V) region is much higher than in the PN ( V rg =12 V, V lg =7 V) region, suggesting the formation of a junction diode when the gates are biased with opposite polarities. To confirm that the asymmetry in the current is because of the formation of a PN or NP junction, we repeat the measurement at negative bias ( Fig. 3b ). Again, the NN and PP regions show the highest current. However, the current in the NP configuration is now much smaller than the current in the PN configuration, confirming the formation of a junction diode as different types of charge carriers are accumulated in the channel. The origin of the strong current modulation induced by the local gates can be explained by the band diagrams in Fig. 3c . In the NN and PP regions, the electric field generated by the two gates is homogeneous and favours either electron (NN) or hole (PP) conduction. As the gates are biased in opposite polarities (PN or NP configuration), a strong horizontal electric field is also present in the b-P region bridging the gates. This large horizontal electric field contributes to charge accumulation in the two different regions of the b-P flake, giving rise to an asymmetric energy landscape. Therefore, the horizontal electric field generated by the local gates and the charge accumulation in the different regions of the b-P flake generate a PN or an NP junction, which is then responsible for the measured rectifying output characteristics ( Supplementary Fig. 5 ) This is similar to a PN junction in bulk-doped materials in which the dopant charges are now located at the surface of the gates rather than in the bulk of the semiconductor itself. The control of the electrical response of the device with the local gates is even more evident by looking at the measured output characteristics in the different doping configurations ( Fig. 3d ). In the NN and PP configurations, the I ds – V ds curves are linear, as expected from Fig. 2b,c . In the PN and NP configurations, the I ds – V ds curves are highly non-linear and the device shows rectifying behaviour, whose direction can be controlled by the gate bias polarity. In the PN configuration, the reverse-bias current is in the order of 1 nA ( V ds =−500 mV), while the reverse-bias current in the NP configuration is ~5 nA ( V ds =500 mV). Photovoltaic effect in locally gated b-P PN junctions To extract the diode parameters, we fit the I ds – V ds curves to a modified version of the Shockley equation that includes parasitic resistances in parallel and in series to the junction (see Supplementary Note 1 ) [30] . The results are summarized in Supplementary Fig. 6 and Supplementary Table 1 . The ideality factors and the series resistances are comparable to PN junctions based on single-layer WSe 2 (refs 31 , 32 ). However, our devices show lower values for the parallel resistance that model the non-zero reverse-bias current. We can attribute this to leakage current due to thermally excited carriers. Given the small bandgap of few-layer b-P, the leakage current is higher than in PN junctions based on larger-bandgap single-layer WSe 2 (refs 31 , 32 ). A useful feature of PN junctions is the large built-in electric field that can be used to separate photoexcited carriers via the photovoltaic effect [31] , [32] , [33] . Upon illumination, the internal electric field at the junction separates photogenerated carriers and gives rise to a photocurrent at zero external bias (short-circuit current, I sc ) and a photovoltage with no current flowing (open-circuit voltage, V oc ). 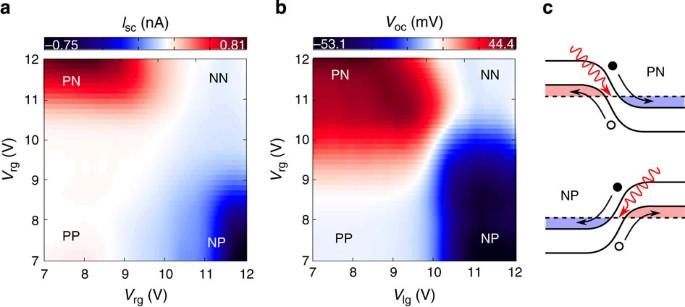Figure 4: Photovoltaic effect in a few-layer black phosphorus PN junction. (a) False-colour map of the short-circuit current (Isc,Vds=0 V) as the voltages on the two local gates are changed independently. (b) False-colour map of the open-circuit voltage (Voc,Ids=0 A) as the voltages on the two local gates are changed independently. (c) Band diagrams illustrating the photovoltaic mechanism in PN and NP configurations: an impinging photon (red arrow) generates an electron–hole pair that is swept away from the junction region by the built-in electric field. (PP:Vlg<8 V,Vrg<10 V, NN:Vlg>8 V,Vrg>10 V, NP:Vlg>8 V,Vrg<10 V, PN:Vlg<8 V,Vrg>10 V). Figure 4a shows a false-colour map of I sc of the device under illumination ( λ =640 nm, P =3.9 μW) as the gate voltages are swept independently. Four regions are clearly visible: high photocurrent in PN and NP configurations and no photocurrent in the PP and NN configurations. Figure 4b displays the measured photovoltage ( V oc ); again, four distinct regions appear: high V oc in PN and NP configurations and zero V oc in PP and NN configurations. The photocurrent and photovoltage are only generated when the local gates are oppositely biased, indicating that the mechanism is photovoltaic originating from the formation of a PN or NP junction in the channel. Figure 4c shows schematically that when the gates are biased in opposite polarities, the internal electric field in the b-P channel separates photogenerated carriers under above-bandgap illumination, generating a photocurrent. If the circuit is kept open, the photogenerated carriers accumulate in distinct parts of the flake, giving rise to a photovoltage. This demonstrates that the b-P PN junction can be used for energy harvesting. Figure 4: Photovoltaic effect in a few-layer black phosphorus PN junction. ( a ) False-colour map of the short-circuit current ( I sc , V ds =0 V) as the voltages on the two local gates are changed independently. ( b ) False-colour map of the open-circuit voltage ( V oc , I ds =0 A) as the voltages on the two local gates are changed independently. ( c ) Band diagrams illustrating the photovoltaic mechanism in PN and NP configurations: an impinging photon (red arrow) generates an electron–hole pair that is swept away from the junction region by the built-in electric field. (PP: V lg <8 V, V rg <10 V, NN: V lg >8 V, V rg >10 V, NP: V lg >8 V, V rg <10 V, PN: V lg <8 V, V rg >10 V). Full size image In Fig. 5a , we characterize the optoelectronic properties of few-layer b-P junction diodes by measuring the output characteristics under illumination with varying incident power ( Fig. 5a ). As the power is increased, the I ds – V ds characteristics shift towards more negative current values. This is consistent with a photocurrent generation mechanism where the separation of the electron–hole pairs is driven by the internal electric field at the junction region: the photocurrent has the same sign as the reverse-bias current; therefore, under illumination and reverse bias, the total measured current is larger than in dark. Thus, an additional forward bias is required to compensate the photogenerated reverse current, giving rise to a non-zero open-circuit voltage. The measured I sc is in the order of 1 nA and V oc ~50 mV at the highest incident power and both I sc and V oc are linear as functions of the incident power ( Supplementary Fig. 7 ). Moreover, we can evaluate the electrical power harvested by the b-P PN junction by ( Fig. 5a , inset) and find that the maximum P el is in the order of 13 pW, in good comparison with other electrostatically defined PN junctions based on WSe 2 (refs 31 , 32 ). The results for other studied devices are shown in Supplementary Figs 8 and 9 ). 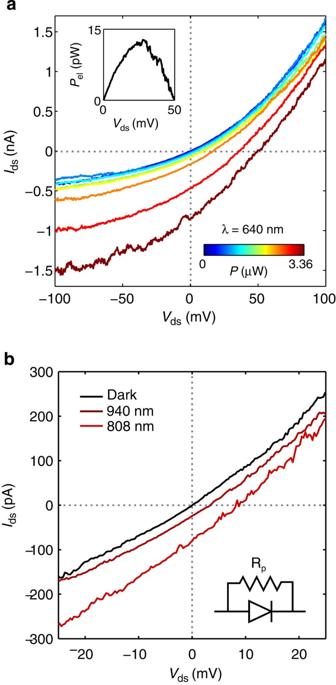Figure 5: Energy harvesting and photodetection as functions of incident power and wavelengths. (a) Output characteristics in the PN configuration as a function of the incident optical power (λ=640 nm). The inset shows the electrical power that can be harvested at the maximum employed illumination power. (b) Output characteristics in the PN configuration in dark (black solid line) and under illumination of different excitation wavelength at fixed power (P=0.33 μW). The inset shows the schematics of the equivalent circuit. Figure 5: Energy harvesting and photodetection as functions of incident power and wavelengths. ( a ) Output characteristics in the PN configuration as a function of the incident optical power (λ=640 nm). The inset shows the electrical power that can be harvested at the maximum employed illumination power. ( b ) Output characteristics in the PN configuration in dark (black solid line) and under illumination of different excitation wavelength at fixed power ( P =0.33 μW). The inset shows the schematics of the equivalent circuit. Full size image While the photocurrent is in the same order of magnitude as similar devices realized with single-layer WSe 2 (refs 31 , 32 ) the open-circuit voltage is lower, due to the smaller bandgap of few-layer b-P. We note that the measured V oc is significantly lower than the predicted bandgap of few-layer b-P (~300 meV). We attribute this to a resistance in parallel ( R p ) to the junction (see inset of Fig. 5b ) which limits V oc by leakage of photogenerated carriers across the junction. The slope of the I ds – V ds curve at V b =0 V (in dark, Fig. 5b ) is a signature of this parallel resistance. The b-P PN junctions show photovoltaic effect up to the NIR part of the electromagnetic spectrum. Figure 5b plots the I ds – V ds curves in the PN configuration in dark (solid black line) and with excitation wavelengths of 808, 885 and 940 nm ( P =0.33 μW). The full data set is presented in Supplementary Fig. 10 and results for another device are presented in Supplementary Fig. 11 . Under illumination, the output characteristics confirm that the photocurrent generation mechanism is dominated by the photovoltaic effect. As the photon energy is increased, both I sc and V oc increase, consistent with increased absorption in the b-P flake at shorter wavelengths. The measured photovoltaic effect up to 940 nm illumination indicates that the bandgap of the b-P flake is smaller than 1.31 eV and demonstrates energy harvesting in NIR part of the spectrum. This constitutes a strong advantage with respect to other 2D semiconductors such as Mo- or W-chalcogenides whose large bandgap (>1.6 eV) limits their applicability in the NIR [13] , [15] , [34] . To further evaluate the performance of the devices, we calculate figures-of-merit such as the fill factor, the external quantum efficiency (EQE; Supplementary Tables 2 and 3 ) and time response ( Supplementary Fig. 12 ). We compare the EQE values to those of PN junctions based on single-layer WSe 2 (ref. 32 ) and find that the EQE for our devices is lower for 532 nm illumination and larger for longer wavelengths ( Supplementary Fig. 13 ). We have fabricated PN junctions based on van der Waals heterostructures of two different 2D materials: h-BN as gate dielectric and b-P as ambipolar semiconducting channel material. We demonstrate full electrostatic control of the device by means of local gating that allows us to tune the electrical behaviour of the device from metallic to rectifying. We observe a strong photocurrent and a significant open-circuit photovoltage, which we attribute to electron–hole separation at the PN junction from the photovoltaic effect, which extends even up to the NIR. Our work sets the ground for further research towards broad-band energy-harvesting devices based on few-layer b-P. Fabrication of b-P PN junctions Vertical heterostructures of h-BN and b-P were fabricated by means of an all-dry transfer technique, as described in refs 18 , 35 We start from a pre-patterned SiO 2 (285 nm)/Si substrate with a pair of split gates (Ti/AuPd 5 nm/60 nm) fabricated by e-beam lithography. We then exfoliate h-BN from a powder (Momentive, Polartherm grade PT110) on a viscoelastic stamp (GelFilm by GelPak) with blue Nitto tape (Nitto Denko Co., SPV 224P). Thin h-BN flakes are identified by optical inspection and stamped on the split gate pair by gently pressing the viscoelastic stamp surface against the substrate and then slowly releasing it. Afterwards, few-layer b-P flakes are identified by the same method and transferred on top of the h-BN flake. The leads (Ti—2 nm/Au—60 nm) are then patterned with e-beam lithography ( Vistec, EBPG5000PLUS HR 100 ), metal deposition ( AJA international ) and lift-off (warm acetone). Atomic force microscopy (AFM) is used to determine the thickness of h-BN and b-P flakes. The AFM ( Digital Instruments D3100 AFM ) is operated in amplitude modulation mode with Silicon cantilevers (spring constant 40 N m −1 and tip curvature <10 nm) to measure the topography and to determine the number of b-P layers. Optoelectronic characterization All the optoelectronic characterization is performed in a Lakeshore Cryogenics probe station at room temperature under vacuum (~10 −5 mBar). The light excitation is provided by diode-pumped solid-state lasers operated in continuous wave mode (CNI Lasers). The light is coupled into a multimode optical fibre (numerical aperture=0.23) through a parabolic mirror ( f reflected =25.4 mm). At the end of the optical fibre, an identical parabolic mirror collimates the light exiting the fibre. The beam is then directed into the cryostat. The beam spot size on the sample has a diameter of 230±8 μm for all wavelengths. The power quoted in the main text is the power incident on the device area ( P ) calculated as follows , where P laser is the power of the laser, A device is the area of the device and A spot is the area of the laser spot. How to cite this article: Buscema, M. et al. Photovoltaic effect in few-layer black phosphorus PN junctions defined by local electrostatic gating. Nat. Commun. 5:4651 doi: 10.1038/ncomms5651 (2014).